Mechanical surface waves accompany action potential propagation Many diverse studies have shown that a mechanical displacement of the axonal membrane accompanies the electrical pulse defining the action potential (AP). We present a model for these mechanical displacements as arising from the driving of surface wave modes in which potential energy is stored in elastic properties of the neuronal membrane and cytoskeleton while kinetic energy is carried by the axoplasmic fluid. In our model, these surface waves are driven by the travelling wave of electrical depolarization characterizing the AP, altering compressive electrostatic forces across the membrane. This driving leads to co-propagating mechanical displacements, which we term Action Waves (AWs). Our model allows us to estimate the shape of the AW that accompanies any travelling wave of voltage, making predictions that are in agreement with results from several experimental systems. Our model can serve as a framework for understanding the physical origins and possible functional roles of these AWs. For many decades, action potentials (APs) have been measured using electrophysiological methods and understood as electrical signals generated and propagating along the axonal membrane [1] . While measuring and understanding the electrical component of the AP has been the focus of most experimental and theoretical efforts, a large number of experimental studies have shown that the AP is accompanied by fast and temporary mechanical changes. These include changes in axonal radius [2] , [3] , [4] , [5] , [6] , [7] , [8] , [9] , [10] , pressure [4] , [11] , optical properties [12] , the release and subsequent absorption of a small amount of heat [7] and shortening of the axon at its terminus when the AP arrives [13] . Despite this wealth of experimental evidence, the physical basis for the mechanical and thermal signals that accompany the AP remains poorly understood. To our knowledge, there have been no attempts to quantitatively describe the mechanical component of the AP as an electrically driven phenomenon. Here we consider a minimal mechanical model of the axon as an elastic and dielectric tube filled and surrounded with viscous fluid. We show that as the AP passes, changes in charge separation across the dielectric membrane alter surface forces that act on the membrane’s geometry. As we show, these forces lead to co-propagating displacements, which we call action waves (AWs, see Fig. 1 ). 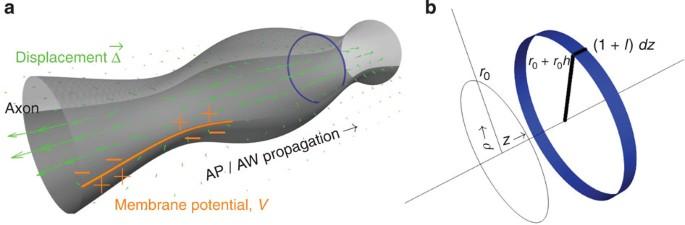Figure 1: Model overview. (a) The action potential and accompanying AW constitute an electromechanical pulse travelling along the axon. The initially depolarized axonal membrane (left, orange + and −) is depolarized as the AP passes (centre). This leads to changes in the electrostatic forces acting on the membrane (grey tube), which drives a co-propagating mechanical surface wave. This surface wave includes a deformation of the axonal surface as well as a displacement of the axoplasmic and extracellular fluid (green arrows). In our model, kinetic energy is carried in the motion of the 3D fluid. (b) Potential energy is stored in deformation of the axonal surface.hdefines a relative height field, andla lateral stretch field, which describe deviations from an unstretched tube of radiusr0as shown in the figure and described in the Results. Figure 1: Model overview. ( a ) The action potential and accompanying AW constitute an electromechanical pulse travelling along the axon. The initially depolarized axonal membrane (left, orange + and −) is depolarized as the AP passes (centre). This leads to changes in the electrostatic forces acting on the membrane (grey tube), which drives a co-propagating mechanical surface wave. This surface wave includes a deformation of the axonal surface as well as a displacement of the axoplasmic and extracellular fluid ( green arrows). In our model, kinetic energy is carried in the motion of the 3D fluid. ( b ) Potential energy is stored in deformation of the axonal surface. h defines a relative height field, and l a lateral stretch field, which describe deviations from an unstretched tube of radius r 0 as shown in the figure and described in the Results. Full size image The electrically driven mechanical modes that we consider are surface waves in which potential energy is stored in the elastic energy associated with deforming the axonal surface, while kinetic energy is carried by the axoplasmic and extracellular fluid, primarily along the direction of propagation. The physics of these modes are governed by the viscosity and density of the axoplasm, the radius of the axon and the elastic moduli of the axonal membrane and cytoskeleton. Our model does not assume a particular mechanism underlying the electrical component of the AP. Indeed, we expect that the surface waves we predict would accompany the AP predicted by Hodgkin and Huxley (HH) and the cable theory, even if they do not contribute to neuronal function. However, our results also allow for the possibility that the mechanical changes that accompany these surface waves feed back and influence the electrical AP, giving them functional importance. Previous models for mechanical aspects of APs have focused on self-sustaining mechanical or electromechanical excitations [14] . Some have considered a nonlinear solitonic excitation [15] , [16] in which a compression wave in the membrane travels at its speed of sound, with a portion of the membrane passing through a reversible freezing transition. Others have considered propagating axoplasmic pressure pulses driven by actomyosin contractility [17] . Here we estimate the displacement and axoplasmic flow field that accompanies and is driven by the electrical AP. We then compare our results with those seen in two experimental systems: the squid giant axon and the garfish olfactory nerve. We also address the issue of thermal changes associated with AP propagation. Finally, we discuss the possible implications of these mechanical waves for neural function. Axons support mechanical surface modes We first define the model shown schematically in Fig. 1 and calculate the susceptibility of displacement fields to time-dependent driving at the axonal surface. In the next subsection, we then estimate the driving force on these modes that accompanies the passing of an AP. Together, these allow us to estimate the AP’s co-propagating displacement field. Axially symmetric flows are described by a time-dependent displacement field (green arrows in Fig. 1a ). We parametrize these using an orthogonal basis, , for the space of axially symmetric and incompressible flows that diagonalizes the vector Laplacian (see Supplementary Note ): where J 0 ( x ) and J 1 ( x ) are Bessel functions of the first kind. We consider the axon to be a tube that, in the absence of displacement, has radius r 0 and that is infinite in extent in the z direction. Many neurons are in a regime where this simplification is reasonable—the garfish nerve is ~20 cm long, and the width of its AP is ~2 mm, roughly 100 × smaller. We assume that the displacement field in the bulk carries the axonal surface along with it, through non-slip boundary conditions. Distortions of this surface can be described by two fields that are entirely determined by Δ: a relative height field h ( z , t )=Δ ρ ( r 0 , z , t )/ r 0 and a lateral stretch field (see Fig. 1b ). These can be expressed in Fourier space, for example, as: In terms of these fields, we can write the kinetic energy and the potential energy as: Where ρ 3D is the density of the bulk fluid, κ is a two-dimensional (2D) compressibility modulus of the axonal surface and where F h/l are externally applied fields. Equations of motion for the bulk field are given by the linearized Navier Stokes equations with each degree of freedom feeling an additional force given by , where the potential energy depends on the Δs through their dependence on h . After Fourier transforming in time, these equations can be combined to yield equations for the Δs in terms of driving forces F and the as yet to be solved for field h (see Supplementary Note ): Integrating the left-hand side of equation (4) according to equation (2) allows us to remove the Δs from the equation and solve for , which are linear in the driving fields and can thus be written as where χ s are susceptibilities. Collecting terms and taking the limit relevant to APs where kr 0 ≫ 1, we can write: where is a Reynolds-like number and where M 11 ( α ) is given by: Notice that this solution for h , in conjunction with equation (4) (and a similar form for χ hl , see Supplementary Note ) allows us to solve for arbitrary Δs, and therefore arbitrary displacement fields induced by driving at the axonal surface. The dispersion relationship for these waves can be extracted from the poles of the susceptibility (equation (5)) and is given by . From the dispersion relation, we can calculate the propagation velocity , which describes the speed at which waves of a given frequency will spread from a point source [18] . When α ≪ 1, as is relevant to most APs in non-myelinated neurons, . When α >>1, as is relevant to the squid giant axon, . We emphasize that the driven waves we consider will travel at the speed of the electrical AP that drives them, c AP , and not at their undriven propagation speed c pr . However, if these speeds are closely matched, then interesting resonant phenomena occur as discussed below. Interestingly, most neurons are in the regime where c pr ~ r 1/2 as predicted by the cable theory. Mechanical modes are driven by charge separation We consider the electrical component of the AP to be a travelling wave of voltage, taking the form , where x = z − c AP t is a co-moving coordinate and c AP is the propagation speed of the AP. Here we take a gaussian form for as plotted in Fig. 2a . The axonal membrane is composed of charged elements that leads to a surface potential on the inner and outer leaflets [19] . As axonal membranes are not symmetrically charged, the potential difference across the membrane is given by where is the difference in surface potentials between the inner and outer leaflets. Throughout, we consider equal to the resting potential for simplicity (see Fig. 2a ), as suggested by the few experiments where it has been measured [19] . As V m changes, the compressive forces on the membrane are altered leading to changes in shape (electrostriction) and corresponding changes in capacitance [19] . 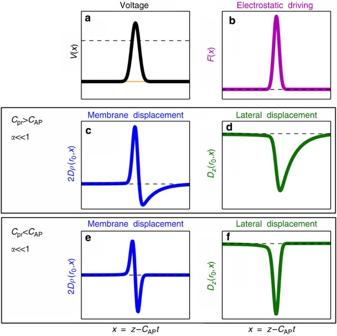Figure 2: Displacements induced by electrical driving. (a) We consider the electrical component of the AP to be a Gaussian wave of depolarization, and take the asymmetry of the surface potential(orange) to be equal to the resting potential. (b) This travelling wave of depolarization leads to a travelling force on the mechanical modes as described in the text. This force leads to a mechanical response that travels alongside the AP as described in the text (c–f). Two components of this wave, the radial displacement of the membrane (c) and the average longitudinal displacement inside of the axon (d), are plotted in the parameter regime whereα≪1 and forcpr>cAP. Ahead of the AP there is a longitudinal displacement backwards relative to the direction of propagation and a slightly inward movement of the membrane. The depolarization of the membrane is accompanied by a swelling and a lowering of the displacement field. After the AP passes, the mechanical modes quickly relax. (e,f) The response to the same driving is shown in the regime whereα≪1 andcpr<cAP. Figure 2: Displacements induced by electrical driving. ( a ) We consider the electrical component of the AP to be a Gaussian wave of depolarization, and take the asymmetry of the surface potential (orange) to be equal to the resting potential. ( b ) This travelling wave of depolarization leads to a travelling force on the mechanical modes as described in the text. This force leads to a mechanical response that travels alongside the AP as described in the text ( c – f ). Two components of this wave, the radial displacement of the membrane ( c ) and the average longitudinal displacement inside of the axon ( d ), are plotted in the parameter regime where α ≪ 1 and for c pr > c AP . Ahead of the AP there is a longitudinal displacement backwards relative to the direction of propagation and a slightly inward movement of the membrane. The depolarization of the membrane is accompanied by a swelling and a lowering of the displacement field. After the AP passes, the mechanical modes quickly relax. ( e , f ) The response to the same driving is shown in the regime where α ≪ 1 and c pr < c AP . Full size image The charge density at the membrane is given by q m ( r )= C 0 V m ( z ), where C 0 is the capacitance per unit area of the unstretched membrane. Here we allow the shape of the membrane to vary at fixed charge per unit membrane. To calculate the resulting forces on the membrane’s geometry we use r ( z )= r 0 (1+ h ( z )), while the length of an infinitesimal cylinder of membrane is given by (1+ l ( z ))d z (see Fig. 2b ). We can estimate the capacitance of this infinitesimal cylinder of membrane C ( z ) dz by taking the membrane to be incompressible in three dimension (3D), and by further assuming that it is an isotropic material so that its capacitance per unit area is inversely proportional to the membrane thickness. (This approximation likely underestimates the effect of electrostriction [20] .) In this approximation C ( z )d z =2 π (1+ h ( z )) r 0 C 0 (1+ l ( z ))d z . The capacitive energy stored in the membrane is thus given by: Including this in the potential energy defined in equation (3), we see that . Specializing to a travelling wave of voltage, , . This driving force is plotted in Fig. 2b . This driving only activates modes for which ω = c AP k , and therefore the AP is accompanied by a co-moving displacement field, , where again x = z − c AP t . Although the mechanical response always travels in a co-moving frame with the electrical component driving it, many of its properties are determined by whether the mechanical propagation speed c pr is faster, slower or comparable to c AP at relevant wavelengths. In Fig. 2 we show two components of the displacement field. First, the membrane displacement, ( Fig. 2c,e ), as observed in experiments that measure axonal swelling, and second, the average lateral displacement inside of the axon, ( Fig. 2d,f ). These are plotted versus x for the case where α ≪ 1 both for c pr > c AP ( Fig. 2c,d ) and for c pr < c AP ( Fig. 2e,f ). Thermal effects arise from the electromechanical wave Previous authors have investigated heat production during AP propagation experimentally [7] , [21] , [22] , [23] in the garfish olfactory nerve, finding the APs depolarization associated with a small release of heat and its repolarization associated with absorption of heat of comparable magnitude. We consider two sources of heating that we expect to accompany AP propagation. First, the HH equations already predict heat production with a similar qualitative shape to that seen in experiments [24] . The sodium influx associated with depolarization is exothermic. Na + ions travel down their concentration and potential gradients so that as the membrane depolarizes the capacitive energy stored in the membrane is released as heat. However, the efflux of K + ions is endothermic, with K + ions travelling up their potential gradients but down their concentration gradients, converting heat in the environment into capacitive energy at the membrane. Thus the HH model predicts that in total, no heat is produced as the AP passes—APs are driven entirely by the entropy of mixing. At the peak of the AP, given a membrane capacitance of 1 × 10 6 F cm −2 (ref. 25 ), the discharging of 70 mV associated with the AP is expected to release approximately of electrical energy as heat. Our model predicts an additional contribution to the heat production associated with AP propagation that arises from the assumed isothermal distortion of the membrane as the AW passes. We assume this process is approximately isothermal because the membrane’s intrinsic time constant is much faster than the ms timescales associated with the AP. This assumption could be called into question if the membrane is near to a phase transition [26] where its equilibration might acquire a hierarchy of longer timescales. In the absence of driving, the membrane’s geometry locally minimizes the free energy so that . In equilibrium, an entropic force stretching the membrane balances an energetic force pulling the membrane in, each of magnitude Tακ where α is the thermal expansion coefficient of the membrane defined by d A / A = α d T . Thus, our theory predicts an additional release of mechanical energy as heat . We ignore two much smaller sources of heating: viscous heating from the flow of axoplasm itself, and a coupling of our height field to V 2 through the changing capacitance. Model predictions agree with experiments We first consider the squid giant axon whose mechanical response has been considered experimentally in refs 9 , 10 , 27 . To quantitatively compare with these experimental results, we use our model described above with parameters from ref. 10 for the squid’s AP speed, c AP =21.2 m s −1 , AP width of 20 mm ( Fig. 3a ) and axonal radius r 0 =238 μm. Although the mechanical properties of the squid giant axon’s sheath and cytoskeleton are not known quantitatively enough for our purposes, we use κ =300 J m −2 for the relevant stretch modulus, which is in the regime expected for the 10-μm sheath of connective tissue surrounding the squid giant axon [28] presuming the sheath has a 3D Young’s modulus around 1 GPa [29] . This choice puts our model into the regime where c pr > c AP . In all of our results, we take the viscosity of axoplasm η to be three times the viscosity of water [30] and assume that the density of the medium ρ 3D =10 3 kg m −3 is that of water. Our model’s prediction for the membrane’s displacement are shown in Fig. 3h in agreement with both the size and shape of the mechanical response seen in ref. 10 . We also plot the average lateral displacement in Fig. 3i that is a novel prediction of our model, which has not been directly measured. 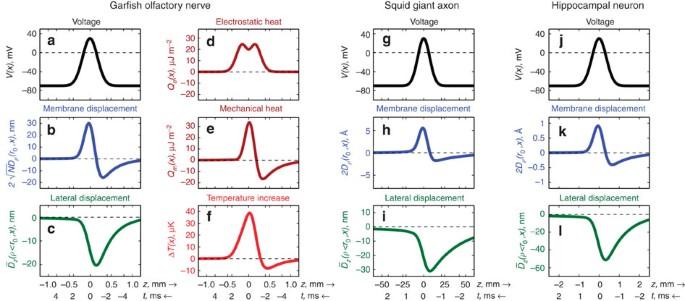Figure 3: Predictions for model systems. Quantitative comparison with three experimentally favoured systems using model and parameters as described in the text. (a,g,j) Voltage: for each, we take as input the shape of the electrical component of the AP as well as its speed from the experimental literature. Displacement: using these in conjunction with our model we make predictions for the membrane displacements (b,h,k) and lateral displacements of the axoplasm (c,i,l). Heat: for the Garfish olfactory nerve, we also consider thermal effects. We plot the electrostatic heat (d) released by the depolarization associated with the AP, the mechanical heat (e) released by the distortion associated with the AW, as well as a prediction for the experimentally observable total heating (f). Figure 3: Predictions for model systems. Quantitative comparison with three experimentally favoured systems using model and parameters as described in the text. ( a , g , j ) Voltage: for each, we take as input the shape of the electrical component of the AP as well as its speed from the experimental literature. Displacement: using these in conjunction with our model we make predictions for the membrane displacements ( b , h , k ) and lateral displacements of the axoplasm ( c , i , l ). Heat: for the Garfish olfactory nerve, we also consider thermal effects. We plot the electrostatic heat ( d ) released by the depolarization associated with the AP, the mechanical heat ( e ) released by the distortion associated with the AW, as well as a prediction for the experimentally observable total heating ( f ). Full size image We next consider the garfish olfactory nerve bundle, which is around 1 mm in diameter and contains approximately N =10 7 non-myelinated axons each of radius r 0 ≈0.125 μm and with a total length of 20 cm [31] . We use the speed of AP propagation to be c AP =0.2 m s −1 and the width of the AP to be 0.4 mm [8] ( Fig. 3a ). We use κ =1 J m −2 in the range suggested by results showing periodic actin rings with a periodicity of ~180 nm [29] , [32] . This is chosen primarily so as to stay in the regime where c pr > c AP . To compare with experimental results in ref. 8 , we assume that each axon swells independently, so that the observed response is . This total response of the nerve is plotted in Fig. 3b , which can be compared with experimental results in refs 7 , 8 . We also predict a lateral displacement in the axon ( Fig. 3c ), which has not been measured, although a shortening of the axon of comparable magnitude, roughly coincident with AP arrival that has been seen in Crab motor neurons [13] . We also compare model predictions to thermal measurements made in the garfish olfactory nerve, where the 10 7 axons contain roughly 6 × 10 4 cm 2 of membrane per cm 3 of volume [31] . As described in the previous section, the HH model already predicts that the activation of all of these nerves at once will lead to the release of electrical energy as heat as plotted in Fig. 3d . Using Tακ =1 J m −2 , our model predicts that the AW releases an additional and similarly sized amount of mechanical energy as heat as shown in Fig. 3e . Thermal diffusivity of water is around 10 5 μm 2 s −1 , so that on the ms timescales relevant to the AP, these very thin (~10 −1 μm) and densely packed axons should have a roughly uniform temperature. Thus, for our calculations, we assume that all of the heat released during the AP is absorbed by a bulk substance with the heat capacity of water. This allows us to predict that a precise and instantaneously equilibrated thermometer would measure a small heating and subsequent cooling as shown in Fig. 3f . Finally, we make predictions for unmyelinated rat hippocampal neurons using r 0 =1 μm, c AP =1 m s −1 and κ =1 J m −2 . Our results, plotted in Fig. 3j–l , are new predictions of our model that could be tested in the near future. Here we have presented a biophysical model for a mechanical AW that accompanies the electrical component of the AP. In our model, electrical driving excites surface waves in which potential energy is stored at the axonal surface and kinetic energy is carried by the bulk fluid. While the mechanical properties of these waves depend on many biophysical parameters discussed below, our model is already in agreement with a range of experimental results [5] , [6] , [7] , [8] , [9] , [13] . The vast majority of theoretical and experimental efforts in neuroscience have been aimed at understanding the electrical component of the AP. The primary focus of this paper is orthogonal: to understand the mechanical component as driven by the well-characterized electrical component of the AP. Our model does not require an underlying theory of how this electrical component arises. We emphasize that any travelling electrical wave will induce a co-propagating mechanical wave, whether arising from an HH-like underlying mechanism or one involving feedback from the mechanical wave itself. Our model differs from most other models of the mechanical response existing in the literature, in that it is electrically driven by the depolarization wave that forms the AP. Where driving has been explicitly considered, it has been taken to arise from actomyosin contractility [17] . While we cannot rule out a possible role for actomyosin contractility as is certainly relevant in cardiomyocytes [33] , the magnitude of the experimentally observed mechanical response does not require extra driving of this form. Our model also differs in the nature of the modes involved. Previous authors [15] , [34] have considered a nonlinear sound wave at the peak of which the membrane has undergone a 2D freezing transition. These authors assume that this solitonic wave independently propagates without dissipation and therefore does not require a continuous input of energy from electrical driving. In our model, only potential energy is stored at the axonal surface, while kinetic energy is carried by the bulk fluid. In refs 15 , 34 , both kinetic and potential energy are stored in the membrane itself. Thus displacements in the axoplasm are a prediction of our model distinct from that in refs 15 , 34 . Our model assumes that, since these displacements are relatively small, we can assume that modes are in the linear response regime. This is in contrast to refs 15 , 20 , 34 in which mechanical nonlinearities, rather than electrical ones, are responsible for the solitonic shape of the AP. Our model makes very different predictions for the thermal signatures that accompany the AP. One prediction of refs 15 , 34 is that the AP should be accompanied by a very large thermal response arising from the latent heat of melting. We predict a much smaller heat signature arising from two distinct mechanisms; the release and subsequent absorption of capacitive energy as heat, and mechanical heat from the stretching of the membrane in the almost isothermal regime. This smaller heat signature is a key prediction distinguishing our model from refs 15 , 34 . The mechanical modes we consider are similar to those studied experimentally in ref. 35 who look at the propagation of surface waves in lipid monolayers at the air–water interface. While these experiments provide inspiration for our model, there are important differences. In addition to using monolayers rather than bilayers, the planar geometry used in ref. 35 leads to qualitatively different dispersion relations and mechanical properties. The same group has recently shown that monolayers also support a second, qualitatively different type of excitation more akin to a 2D sound wave propagating in the membrane, with subtle and intriguing nonlinear properties [36] . These modes are absent entirely from our model, as we assume that the membrane and surrounding fluid are incompressible in 3D. However, we cannot rule out their relevance in real neurons. Much of the uncertainty in our model arises from our uncertain knowledge of the elastic properties of the axon, which are determined by a combination of the elastic properties of the axonal membrane and the architecture of the axonal cytoskeleton, each being the focus of intense inquiry [32] , [37] , [38] , [39] . The axoplasmic membrane and associated cytoskeletal fibres make up the axonal surface, which contributes to the elastic energy of deformations through surface terms. These enter our model in terms of the 2D displacement fields h and l . The membrane contributes a term that punishes stretching through elastic modulus κ 2D , which multiplies in the potential energy . It also contributes a term that punishes changes in total area through tension σ ,which multiplies in . This term is subdominant in the regime where kr 0 ≪ 1, and so we drop it here. Recent experiments have demonstrated that the axonal membrane cytoskeleton is exquisitely ordered, forming a quasi-one-dimensional lattice, with evenly spaced actin rings [32] . These likely contribute a term to the potential energy that depends only on the height field h , motivating our choice of potential energy in equation (3). The same study found longitudinal spectrin fibres, which likely contribute a term to the potential energy proportional to . The bulk of the axon contains microtubules [38] , which are arranged parallel with the axons. The present analysis focuses on the elastic properties of the surface, assuming that the bulk is purely viscous, with little elastic resistance to shear. This is motivated by the parallel microtubule arrangement within the axon, which should lead to a very anisotropic shear modulus. In our model, the dominant shears are orthogonal to the energetically unfavourable directions. Thus, while it is possible that the bulk elasticity makes important contributions to mechanical properties relevant for the AW, we ignore them here. Our finding that mechanical AWs of the size and shape seen experimentally naturally accompany the electrical AP suggests the possibility that AWs might exist even without functional significance. On the other hand, it seems likely that biology would take advantage of this co-propagating information, especially if real neurons are indeed in the regime where c pr > c AP in which the mechanical component arrives before the electrical AP. We discuss several mechanistic possibilities. AWs could feed back and influence the electrical component of the AP. Such a picture is broadly supported by experiments that see changes in electrical properties and even the triggering of APs on mechanical stimulation of single neurons [40] , [41] , [42] . Furthermore, particular cell types are known to have important electromechanical coupling, most notably cardiac cells [43] and stereocilia of the inner ear [44] . Intriguingly, these stereocilia sense excitations of similar surface waves propagating in the cochlea, albeit in a very different geometry. Mechanics could influence electrical properties by direct alteration of membrane conductance and/or capacitance or by influencing the gating of voltage-gated ion channels. Studies in artificial lipid bilayers without protein channels have shown ion channel-like conductances sensitive to stretching, although their existence in neuronal membranes and relevance to the AP has not been established [16] , [45] , [46] . Membrane mechanical properties are also known to influence some ion channels directly [47] , including the voltage-gated sodium channels responsible for the AP [48] , [49] . We consider two ways in which channels could acquire mechanical sensitivity. First, a channel could sense membrane tension by changing its 2D membrane footprint by Δ A upon activation. Such a channel would have its gating altered substantially by changes in tension greater than k B T /Δ A (ref. 47 ). The Large-Conductance Mechanosensitive Channels (MscL) channel, a bacterial osmotic pressure sensor for which Δ A ~20 nm, can detect changes in tension smaller than 10 −3 N m −1 (ref. 47 ), while measured mechanosensitivity of Na channels is smaller, with a change in tension closer to 10 −2 N m −1 required [49] . Our model predicts changes in tension of order κ 2D ( l + h )~10 −4 N m −1 , close to the limit of sensitivity for dedicated tension sensors, but likely irrelevant for Na channel function. More plausibly relevant for the AP, a channel could directly sense displacements by connecting to a cytoskeletal element through a tether whose length is coupled to channel activity [50] . Such a mechanism is thought to convert mechanical signals in the inner ear into electrical ones, where channels can sense displacements of 5-μm hair cells by as little as 0.3 nm, about as large as the radial displacements predicted by our model for typical neurons, and much smaller than the horizontal ones. Although this mechanism remains speculative even in the inner ear, Na channels do coordinate at nanometric scales with periodic actin rings and spectrin [32] . Na channels are anchored to the cytoskeleton by ankyrin-G, which is homologous to the ankyrin repeats in specialized transient receptor potential (TRP) channels widely believed to play the role of the mechanical to electrical transducer in the inner ear [51] . Both membrane-mediated currents and stretch regulation of ion channels could be especially sensitive near a 2D liquid–gel transition [46] or a liquid–liquid critical point, as seen experimentally in vesicles taken from a mammalian cell line [26] . Our model adds to a more complete theory for AP generation and propagation that explains electrical, mechanical, chemical and thermal aspects. We hope this more complete theoretical understanding of the phenomena accompanying the AP will guide experiments seeking to understand the role of the striking cytoskeletal ultrastructure recently available to state-of-the-art super-resolution techniques [32] , [39] . We foresee future theoretical and experimental work will highlight the extent to which AWs play a functional role in neuronal information processing. Numerical methods Calculations were performed in two steps in Figs 2 and 3 . First, functions M ( α ) (defined in equation (6) and in Supplementary Note ) were numerically estimated using Mathematica, at 400 logarithmically spaced points covering the relevant range. We used this as a smooth function by linearly interpolating between these points in log-space, leading to very small numerical errors. These functions were used in python to calculate the susceptibility as a function of wavelength and frequency according to equation (5). Utilizing these functions and standard Fourier transform techniques, we numerically estimated co-propagating mechanical and thermal aspects according to the equations described in the Results. How to cite this article: El Hady, A. and Machta, B. B. Mechanical surface waves accompany action potential propagation. Nat. Commun. 6:6697 doi: 10.1038/ncomms7697 (2015).